Mitochondrial function and lifespan of mice with controlled ubiquinone biosynthesis Ubiquinone (UQ) is implicated in mitochondrial electron transport, superoxide generation and as a membrane antioxidant. Here we present a mouse model in which UQ biosynthesis can be interrupted and partially restored at will. Global loss of UQ leads to gradual loss of mitochondrial function, gradual development of disease phenotypes and shortened lifespan. However, we find that UQ does not act as antioxidant in vivo and that its requirement for electron transport is much lower than anticipated, even in vital mitochondria-rich organs. In fact, severely depressed mitochondrial function due to UQ depletion in the heart does not acutely impair organ function. In addition, we demonstrate that severe disease phenotypes and shortened lifespan are reversible upon partial restoration of UQ levels and mitochondrial function. This observation strongly suggests that the irreversible degenerative phenotypes that characterize ageing are not secondarily caused by the gradual mitochondrial dysfunction that is observed in aged animals. Ubiquinone (UQ), also known as coenzyme Q (CoQ), is a redox-active lipophilic molecule that is found in all cells and in the membranes of many organelles where it participates in a variety of cellular processes [1] . In the inner membrane of mitochondria, UQ diffuses freely and is necessary for the function of the electron transport chain (ETC), as it enables the transfer of electrons from mitochondrial complexes I and II to mitochondrial complex III (ref. 2 ). Thus, UQ is necessary for appropriate mitochondrial ATP generation. UQ is also believed to be critically involved in mitochondrial ROS generation, as the UQ ·− ubisemiquinones generated during electrons transport can react with molecular oxygen to form the superoxide anion [3] , [4] . In its reduced form, UQ has been suggested to be an effective antioxidant, protecting cellular membranes from lipid peroxidation [5] . It is of note, however, that many of these properties of UQ were studied in vitro by biochemical techniques but were not always formally established in vivo , as adequate animal models with controlled level of UQ were not previously available. UQ has an aromatic head group and a polyisoprenoid side chain varying in length between species. The side chain comprises 10 subunits in humans (UQ 10 ) and 9 in mice (UQ 9 ), where UQ 10 is also present as a minor species. The biosynthetic pathway of UQ has been evolutionarily conserved. It requires at least 10 separate proteins in vertebrates, termed prenyl diphosphate synthase (PDSS) and COQ proteins [6] . The long isoprenoid side chain is synthesized by PDSS and subsequently attached to carbon C3 of the aromatic ring of 4-hydroxybenzoic acid (4-HB) by the COQ2 prenyl transferase ( Fig. 1a ). The remainder of the pathway serves to modify the ring to yield UQ. In particular, carbon C5 and C6 are each hydroxylated, with a subsequent methylation step yielding methoxyl groups. The conserved enzyme that is required for the hydroxylation of C6 is named Coq7p in yeast, CLK-1 in Caenorhabditis elegans , MCLK1/COQ7 in mice (subsequently called MCLK1) and COQ7 in humans. It converts demethoxyubiquinone (DMQ) to hydroxyubiquinone, which is then turned into UQ by the COQ3 enzyme. Mutants missing the enzyme do not produce UQ but instead accumulate the biosynthetic precursor DMQ [7] , [8] , [9] . A yeast study showed that treatment of a coq7 null mutant with 2,4-dihydroxybenzoic acid (2,4-DHB) results in restoration of UQ 6 biosynthesis [10] . 2,4-DHB is an analogue of the natural precursor (4-HB) that already carries a hydroxyl group at carbon C6 ( Fig. 1b ), thus restoring UQ synthesis by obviating the need for the missing enzymatic step. 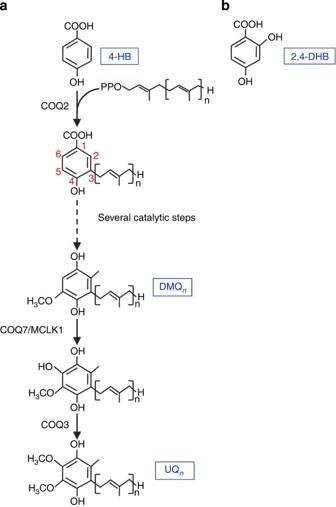Figure 1: The UQ biosynthetic pathway. (a) Schematic overview of the UQ biosynthesis pathway. 4-HB is the aromatic ring precursor of UQ. MCLK1/COQ7 carries out the penultimate biosynthetic step, the hydroxylation of DMQ. (b) Chemical structure of 2,4-DHB. ‘n’ denotes the number of subunits of the isoprenoid side chain. Figure 1: The UQ biosynthetic pathway. ( a ) Schematic overview of the UQ biosynthesis pathway. 4-HB is the aromatic ring precursor of UQ. MCLK1/COQ7 carries out the penultimate biosynthetic step, the hydroxylation of DMQ. ( b ) Chemical structure of 2,4-DHB. ‘ n ’ denotes the number of subunits of the isoprenoid side chain. Full size image In human patients, UQ deficiency due to mutation in a variety of genes [6] , [11] , [12] , [13] , [14] , [15] , [16] , [17] , [18] , [19] is associated with a wide spectrum of clinical symptoms, including nephrotic syndrome, encephalomyopathy, ataxia and Leigh syndrome [12] , [15] , [16] , [20] , [21] . In mice, total knockout (KO) of Mclk1 is embryonic lethal, similar to mutations in other UQ biosynthetic enzymes and other key ETC components [8] , [22] , [23] , [24] , [25] . Loss of one copy of Mclk1 in Mclk1 +/− heterozygous mice is viable but leads to a decrease in UQ 9 levels in the inner mitochondrial membrane, where the committed steps of UQ synthesis are taking place [23] . Mouse cells in which MCLK1 activity is absent are viable in vitro . They essentially lack UQ 9 and show an accumulation of DMQ 9 (refs 8 , 9 , 22 ). However, our recent study with a liver-specific Mclk1 KO strain suggested that DMQ has no activity in UQ-dependent mitochondrial electron transport [9] . Mitochondria and mitochondrial dysfunction hold a prominent place in many theories of ageing. For instance, the oxidative stress theory of ageing suggests that organisms age because of cumulative damage from ROS, in particular mitochondrial ROS, and that mitochondrial proteins and DNA are particularly susceptible to oxidative damage because of their close proximity to the sites of ROS generation [26] . Independently of the origin of the damage, it has been proposed that the progressive accumulation of somatic mutations in mitochondrial DNA (mtDNA) that occurs throughout life induces mitochondrial dysfunction, which in turn participates in causing the ageing process [27] . Consistent with these theories, animal models with various genetic defects in mitochondrial function present with a shortened lifespan and ageing-like phenotypes at an early age [28] . At a purely observational level, many studies have reported degenerative changes in the mitochondria of elderly humans and aged animals, including lower overall functional capacity [27] , [29] , [30] , [31] , [32] . Finally, a number of age-associated diseases have been linked to mitochondrial defects [33] . For all these reasons, mitochondrial dysfunction has been placed among the nine hallmarks of ageing that have been recently formulated [34] . However, in recent years, extensive genetic studies of the ageing process of vertebrates [35] and invertebrates [36] , [37] , in particular C. elegans , have failed to confirm a causative role for mitochondrial dysfunction in ageing. Furthermore, as briefly reviewed above, much of the evidence obtained in vertebrates is correlative in nature or based on shortened lifespans associated with severe irreversible disease states. Here we describe the first mammalian model of controlled UQ biosynthesis. After induced homozygous KO of a floxed Mclk1 gene via a globally expressed tamoxifen (TM)-dependent CreER T2 transgene, adult animals gradually lose UQ and mitochondrial function, thereby leading to a progressively worsening phenotype, which is ultimately fatal. Dietary UQ 10 was almost completely ineffective in rescuing the phenotype of Mclk1 KO mouse mutants, but feeding 2,4-DHB resulted in partial restoration of UQ biosynthesis and mitochondrial respiration, and led to a marked rescue of the mutant phenotype, including lifespan. This suggests that providing unnatural biosynthetic precursors could benefit patients with primary genetic defects in UQ biosynthesis or in other biosynthetic pathways. It also provided us with a method to study previously inaccessible questions about the in vivo functions of UQ and about the role of mitochondrial dysfunction in the ageing process. Adult-onset global Mclk1 KO mice We previously described a conditional (floxed) allele of Mclk1 in which exons 2 and 3 can be excised by Cre recombinase [9] . We combined the floxed Mclk1 allele with a CAG -CreER T2 transgene [38] that expresses a TM-inducible Cre recombinase under the control of the ubiquitous CAG promoter (cytomegalovirus early enhancer/chicken β-actin). At 2 months of age, CAG -CreER T2 ;Mclk1 loxP/loxP mice were treated with TM, thus ablating Mclk1 in a wide variety of tissues (subsequently referred to as adult-onset global Mclk1 KO (aog Mclk1 KO)). 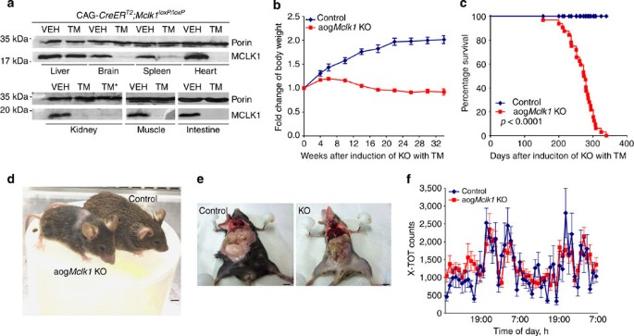Figure 2: Phenotypes of adult-onset globalMclk1KO mice. (a) Western blot analysis of MCLK1 from mitochondrial fractions. MCLK1 was virtually undetectable in heart, kidneys, skeletal muscles, brain, spleen and intestine 2 weeks after the final TM injection. Lanes: VEH: samples from vehicle-administered CAG-CreERT2;Mclk1loxP/loxPmice; TM: samples prepared 2 weeks after completion of TM administration (KO). TM*: samples prepared from 2,4-DHB-treated KO mice after~6 months of treatment. Blot images were cropped for clarity. Some images were rotated so that the vehicle-injected group is on the left. Original western blots are presented inSupplementary Fig. 10. (b) Body weight change curves for control and adult-onset globalMclk1(aogMclk1) KO mice. The differences between control and KO mice were significant from 6 weeks onwards (P<0.05, two-way analysis of variance (ANOVA)/Bonferronipost hoctest).n=7–24. (c) Kaplan–Meier survival curves (n=32).P<0.0001, log-rank test. (d) aogMclk1KO mice showed reduced body size and lower hair density (6 months after KO induction). Scale bars, 1 cm. (e) Representative pictures showing that KO mice have reduced abdominal fat. (f) Normal locomotory activity at 6 months after induction ofMclk1KO. n=9. Data are mean±s.e.m.P=0.54, two-way ANOVA/Bonferronipost hoctest. Figure 2a shows that 2 weeks after completion of TM injections, the MCLK1 protein was virtually absent in most of the organs examined (brain, heart, kidney, muscle, spleen and intestine). Thus, in the presence of TM, Cre/loxP-mediated recombination induced rapid gene inactivation of the floxed Mclk1 alleles in a broad range of tissues. One notable exception was the liver in which the level of MCLK1 protein was not affected ( Fig. 2a ), likely reflecting low expression of the CAG -CreER T2 transgene in this organ, as has been previously reported [38] . Figure 2: Phenotypes of adult-onset global Mclk1 KO mice. ( a ) Western blot analysis of MCLK1 from mitochondrial fractions. MCLK1 was virtually undetectable in heart, kidneys, skeletal muscles, brain, spleen and intestine 2 weeks after the final TM injection. Lanes: VEH: samples from vehicle-administered CAG -CreER T2 ;Mclk1 loxP/loxP mice; TM: samples prepared 2 weeks after completion of TM administration (KO). TM*: samples prepared from 2,4-DHB-treated KO mice after~6 months of treatment. Blot images were cropped for clarity. Some images were rotated so that the vehicle-injected group is on the left. Original western blots are presented in Supplementary Fig. 10 . ( b ) Body weight change curves for control and adult-onset global Mclk1 (aog Mclk1 ) KO mice. The differences between control and KO mice were significant from 6 weeks onwards ( P <0.05, two-way analysis of variance (ANOVA)/Bonferroni post hoc test). n =7–24. ( c ) Kaplan–Meier survival curves ( n =32). P <0.0001, log-rank test. ( d ) aog Mclk1 KO mice showed reduced body size and lower hair density (6 months after KO induction). Scale bars, 1 cm. ( e ) Representative pictures showing that KO mice have reduced abdominal fat. ( f ) Normal locomotory activity at 6 months after induction of Mclk1 KO . n =9. Data are mean±s.e.m. P =0.54, two-way ANOVA/Bonferroni post hoc test. Full size image Following induction of Mclk1 KO by TM, the mice exhibited severe growth retardation ( Fig. 2b ) but survived for almost a full year with a median survival of ~276 days ( Fig. 2c ). From 4 months onwards, KO mice also gradually lost their fur ( Fig. 2d ). At 6 months, KO mice were about half the weight of their vehicle-injected controls, with significantly lower body fat content ( Fig. 2d,e ). The mean absolute weights of many organs (brain, heart, kidneys and skeletal muscles) were lower than in controls, but were actually higher relative to body weight ( Supplementary Fig. 1a,b ). Furthermore, oxygen consumption was elevated when normalized to the weight of four internal organs ( Supplementary Fig. 1c ). The observation of high relative organ weights is consistent with the severe loss of fat tissue ( Fig. 2e ). See below for a discussion of the findings about oxygen consumption. Food intake normalized to body weight was not significantly affected ( Supplementary Fig. 1d ) nor were locomotory activity scores ( Fig. 2f ). In circulating blood, markedly elevated lactate levels were observed 6 months after KO induction. In addition, fasting blood glucose and non-fasting plasma triglycerides were found to be lower in KO mice than in controls ( Table 1 ). Table 1 Blood and plasma measurements from aog Mclk1 KO mice. Full size table Vehicle-injected CAG -CreER T2 ;Mclk1 loxP/loxP mice and TM-injected Mclk1 loxP/loxP mice were phenotypically healthy and are still alive after >2 years, demonstrating that neither TM treatment itself nor the presence of the CreER T2 protein alone has noticeable toxicity on the experimental animals. UQ depletion and respiratory chain dysfunction in aog Mclk1 KO mice Six months after induction of the aog Mclk1 KO, all organs examined except the liver showed substantial loss of UQ along with accumulation of DMQ, with the most severe depletion in heart, kidneys, muscles and intestine ( Fig. 3a ). The level of UQ 9 in the strongly affected tissues averaged only 10–15% of controls. Decreased UQ 9 levels and appearance of DMQ 9 were also observed in quinone extracts from the ears of aog Mclk1 KO mice ( Supplementary Fig. 1e ); thus, hair loss of the mutant mice could be, at least in part, induced by UQ deficit in epidermis and/or hair follicles. We also established a time-course for the changes in quinone levels. A time-dependent, gradual loss of UQ was observed in all the following tissues analysed: heart, kidney, skeletal muscle and intestine, where an ~80% reduction in UQ 9 levels was observed 8–14 weeks after the induction of Mclk1 KO ( Fig. 3b ). Over the next 24–30 weeks, UQ 9 concentrations continued to fall, but to a lesser extent. Overall, UQ was lost at a much slower rate in the Mclk1 KO tissues than expected from its previously estimated 50–125 h half-life [39] . The kidneys and intestine appeared to lose UQ faster than the heart and skeletal muscles ( Fig. 3b ). As a rapid cell turnover would result in fast dilution of the initial UQ pool, tissue renewal rate should be an important parameter determining how fast UQ content is depleted when its biosynthesis is interrupted. Heart and skeletal muscles are composed mainly of post-mitotic, terminally differentiated cells. Comparatively, kidneys and intestines have a relatively higher turnover rate because renal tubular and intestinal epithelia are consistently being renewed by proliferation and differentiation of progenitor cells and/or divisions of differentiated cells. The accumulation of DMQ 9 appeared to mirror that of UQ 9 in controls ( Fig. 3b ), indicating that the biosynthetic pathway upstream of MCLK1 was still active and that DMQ 9 metabolism is similar to that of UQ 9 . Note that the absolute amount of DMQ 9 corresponding to a peak area of high-performance liquid chromatography (HPLC)-ultraviolet absorption is unknown because synthetic DMQ 9 is not available to use as a standard. Thus, there might actually be as much DMQ in the mutants as UQ in the controls. 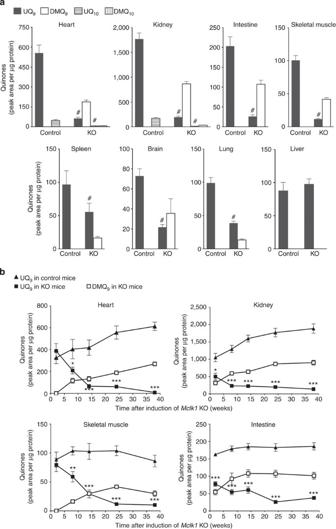Figure 3: Widespread depletion of UQ levels in aogMclk1KO mice. (a) Quinone concentrations in whole-tissue homogenates were measured ~6 months after TM (KO) or vehicle (control) administration. After loss ofMclk1for 6 months, all the tissues examined, except the liver, exhibited a large decrease in UQ9content along with accumulation of DMQ9. UQ10level was also affected as evidenced in the kidneys and heart, where high UQ levels allow the detection of UQ10.n=9–11.#P<0.001 with respect to control groups (Student'st-test). (b) Time-course of tissues UQ levels after loss ofMclk1. n=4−11.*P<0.05, **P<0.05, ***P<0.001 for comparison of UQ9levels between control and KO groups (two-way analysis of variance/Bonferronipost hoctest). Data are shown as peak areas on HPLC chromatograms normalized to protein content (mean±s.e.m.). Figure 3: Widespread depletion of UQ levels in aog Mclk1 KO mice. ( a ) Quinone concentrations in whole-tissue homogenates were measured ~6 months after TM (KO) or vehicle (control) administration. After loss of Mclk1 for 6 months, all the tissues examined, except the liver, exhibited a large decrease in UQ 9 content along with accumulation of DMQ 9 . UQ 10 level was also affected as evidenced in the kidneys and heart, where high UQ levels allow the detection of UQ 10 . n =9–11. # P <0.001 with respect to control groups (Student's t -test). ( b ) Time-course of tissues UQ levels after loss of Mclk1. n= 4−11. *P <0.05, ** P <0.05, *** P <0.001 for comparison of UQ 9 levels between control and KO groups (two-way analysis of variance/Bonferroni post hoc test). Data are shown as peak areas on HPLC chromatograms normalized to protein content (mean±s.e.m.). Full size image We also examined purified mitochondria for UQ depletion. After loss of Mclk1 for 6 months, an 89–93% decrease in UQ levels was seen in kidney and heart mitochondria, along with a substantial accumulation of DMQ ( Fig. 4a ). This magnitude of UQ depletion is similar or superior to that observed in whole-tissue homogenates ( Figs 3a and 4a ). To assess the effect on ETC function, we measured state 3 respiration of freshly isolated mitochondria. Compared with controls, the heart, muscle and kidney mitochondria from KO mice showed a ~50% reduction in state 3 respiration with either complex I or II respiratory substrates ( Fig. 4b ). The respiratory control ratio was mildly decreased ( Supplementary Table 1 ). The ratio of ADP molecules phosphorylated to oxygen atoms reduced (ADP/O ratio), which reflects the efficiency of oxidative phosphorylation, was also only slightly affected ( Supplementary Table 1 ), suggesting that the coupling of phosphorylation to respiration was largely preserved. We used kidney mitochondria for additional measures. The activities of pairs of complexes (I+III or II+III), which rely on endogenous UQ, were drastically decreased, whereas the activities of single respiratory complexes were increased, pointing to partial compensatory upregulation ( Fig. 4c ). The activity of citrate synthase (CS) was also slightly elevated ( Fig. 4c ). Addition of decylubiquinone (a synthetic hydrophilic analogue of UQ) to the reaction mixture increased the activity of the complex pair II+III by ~1.8-fold in the mitochondria from control mice but by ~3.7-fold in mutant mitochondria ( Fig. 4c ), which is consistent with a severe defect in UQ-dependent electron transport in the KO. The increased activities of the individual complexes in the KO mitochondria (mostly a higher activity of complex II) also likely contributes to the greater magnitude of increase in II+III activity after the addition of decylubiquinone. As expected, we observed no changes in mitochondrial UQ content or respiration rates in TM-treated Mclk1 loxP/loxP mice ( Supplementary Table 2 ). 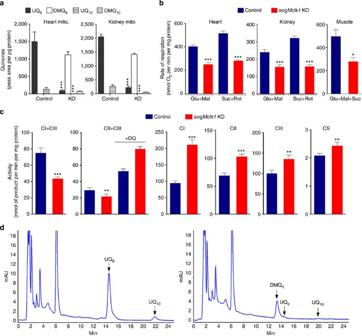Figure 4: Mitochondrial UQ levels, respiration rates and enzyme activities in aogMclk1KO mice. (a) Mitochondrial (mito) quinone levels~6 months afterMclk1KO induction.n=7–9. (b) Mitochondrial oxygen consumption rates (state 3).n=9 for the kidney,n=8 for the heart andn=3 for the skeletal muscle. Glu, glutamate; Mal, malate; Suc, succinate; Rot, rotenone. (c) Activities of respiratory complexes and CS in the kidney mitochondria isolated from ~8-month-old aogMclk1KO or control mice (~6 months after the last dose of TM or vehicle).n=7–11. DQ, decylubiquinone. Values are shown as mean±s.e.m. *P<0.05, **P<0.01, ***P<0.001 versus controls (one-way analysis of variance test for the differences in complex II-III activity data; for all other data, Student’st-test was used). (d) Representative HPLC-ultraviolet chromatograms of quinone extracts from the hearts of control (left) or KO mice (right). Isolation and HPLC analysis of quinones were performed on samples collected from live mice~8 months after vehicle or TM administration was completed. Heart homogenates with 1 mg of protein were used. Figure 4: Mitochondrial UQ levels, respiration rates and enzyme activities in aog Mclk1 KO mice. ( a ) Mitochondrial (mito) quinone levels~6 months after Mclk1 KO induction. n= 7–9. ( b ) Mitochondrial oxygen consumption rates (state 3). n =9 for the kidney, n =8 for the heart and n =3 for the skeletal muscle. Glu, glutamate; Mal, malate; Suc, succinate; Rot, rotenone. ( c ) Activities of respiratory complexes and CS in the kidney mitochondria isolated from ~8-month-old aog Mclk1 KO or control mice (~6 months after the last dose of TM or vehicle). n =7–11. DQ, decylubiquinone. Values are shown as mean±s.e.m. * P <0.05, ** P <0.01, *** P <0.001 versus controls (one-way analysis of variance test for the differences in complex II-III activity data; for all other data, Student’s t -test was used). ( d ) Representative HPLC-ultraviolet chromatograms of quinone extracts from the hearts of control (left) or KO mice (right). Isolation and HPLC analysis of quinones were performed on samples collected from live mice~8 months after vehicle or TM administration was completed. Heart homogenates with 1 mg of protein were used. Full size image Surprisingly, we observed that at ~8 months after Cre induction, before the KO mice started to die, there was hardly any UQ left in the heart ( Fig. 4d ). Thus, the heart is still able to function sufficiently to support life with almost no UQ (at least under non-stress laboratory conditions). Moreover, echocardiographic examination of the heart of mutant and control mice established that, despite a smaller heart size, the KO mice had similar baseline parameters of systolic and diastolic function as controls, including left ventricle relative wall thickness, left ventricle percent fractional shortening, ratio of early to late diastolic mitral flow velocity (E/A ratio) and deceleration time ( Supplementary Fig. 2 ). These findings are particularly intriguing, given that the mammalian heart requires an extraordinary amount of mitochondrial ATP for its contractile function, and it has been generally assumed that energy-demanding tissues such as the heart are highly susceptible to UQ deficit and defective mitochondrial energy metabolism. To test the effect of UQ depletion and mitochondrial dysfunction on the kidney, we performed histological analysis and measured blood urea nitrogen (BUN). We observed normal appearance of kidney glomeruli and tubules in the kidney 6 months after induction of Mclk1 KO ( Supplementary Fig. 3 ). On the other hand, BUN levels were found to be higher in aog Mclk1 KO mice than in controls 9 months after the KO ( Supplementary Table 3 ). These observations suggest that at the end of their life, mutant mice had partially compromised kidney function, but loss of UQ and mitochondrial function for 6 months had no devastating effect on kidney morphology. Lower ROS production by heart mitochondria of aog Mclk1 KO mice As mentioned in the introduction, UQ is closely involved in superoxide generation by the respiratory chain. Using the well-established horseradish peroxidase (HRP)-linked Amplex Red assay, we examined hydrogen peroxide (H 2 O 2 ) production by heart mitochondria from aog Mclk1 KO mice to assess the effect of severe UQ deficiency on net ROS release from mitochondria. We found that UQ depletion significantly decreased H 2 O 2 production in mouse heart mitochondria ( Fig. 5a ). This decrease in net ROS production was observed in nearly all test conditions: (1) with complex I substrates (glutamate plus malate) in the presence of the complex I UQ site inhibitor rotenone; (2) with complex I substrates in the presence of the complex III inhibitor antimycin A (which blocks electrons transport without preventing the formation of ubisemiquinone); (3) with the complex II substrate succinate in the presence of ETC inhibitors; and (4) with succinate without inhibitors. 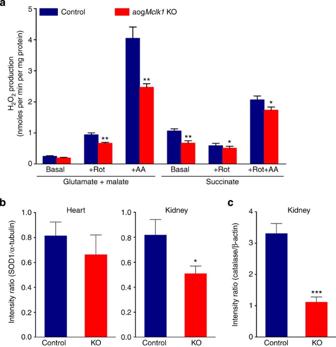Figure 5:H2O2production rate in heart mitochondria and SOD1 and catalase levels. (a) H2O2production rate in isolated heart mitochondria. A low basal H2O2production was seen in presence of complex I substrates (glutamate plus malate) alone. Measurement in the presence of succinate (complex II substrate) detects ROS production from complex I during reverse electron transport. Rotenone (Rot), a UQ site inhibitor at complex I, increases electron leak during the oxidation of complex I substrates, while in succinate-fueled mitochondria it blocks the reverse electron flow and thus decreases ROS production. Inhibition of complex III by antimycin A (AA) resulted in markedly increased generation of superoxide and H2O2. Measurements were performed on intact heart mitochondria isolated at 6 months after KO induction by TM. Bars indicate mean±s.e.m. (n=6 per group). (b) SOD1 protein levels in the heart and kidney of agoMclk1KO mice versus control mice. (c) Catalase protein level in the kidney. Protein extracts were prepared ~6 months after the last dose of TM (KO) or vehicle (control). α-Tubulin and β-actin were used as loading controls. The bar graphs show the ratios of individual band densities divided by the respective loading control densities (n=4). Error bars are s.e.m. The information about the antibodies and the original western blot images can be found inSupplementary Information. *P<0.05, **P<0.01, ***P<0.001 versus respective controls (Student’st-test). Figure 5: H 2 O 2 production rate in heart mitochondria and SOD1 and catalase levels. ( a ) H 2 O 2 production rate in isolated heart mitochondria. A low basal H 2 O 2 production was seen in presence of complex I substrates (glutamate plus malate) alone. Measurement in the presence of succinate (complex II substrate) detects ROS production from complex I during reverse electron transport. Rotenone (Rot), a UQ site inhibitor at complex I, increases electron leak during the oxidation of complex I substrates, while in succinate-fueled mitochondria it blocks the reverse electron flow and thus decreases ROS production. Inhibition of complex III by antimycin A (AA) resulted in markedly increased generation of superoxide and H 2 O 2 . Measurements were performed on intact heart mitochondria isolated at 6 months after KO induction by TM. Bars indicate mean±s.e.m. ( n =6 per group). ( b ) SOD1 protein levels in the heart and kidney of ago Mclk1 KO mice versus control mice. ( c ) Catalase protein level in the kidney. Protein extracts were prepared ~6 months after the last dose of TM (KO) or vehicle (control). α-Tubulin and β-actin were used as loading controls. The bar graphs show the ratios of individual band densities divided by the respective loading control densities ( n =4). Error bars are s.e.m. The information about the antibodies and the original western blot images can be found in Supplementary Information . * P <0.05, ** P <0.01, *** P <0.001 versus respective controls (Student’s t -test). Full size image No increase of oxidative stress in aog Mclk1 KO mice As UQ is believed to be a membrane antioxidant, we characterized overall oxidative stress in mutant mice. We measured plasma concentrations of F 2 -isoprostanes in aog Mclk1 KO mice 8 months after induction of the KO, at a time when they were already displaying marked phenotypes and were close to death. The level of F 2 -isoprostanes in the circulation is a well-accepted biomarker of lipid peroxidation and an index of systemic oxidative stress. We observed no significant difference in plasma F 2 -isoprostane concentration between KO mice and age-matched controls ( Supplementary Fig. 4a ). Similarly, the plasma levels of 8-OHdG, which reflect the degree of oxidative damage to DNA, were found to be indistinguishable from controls ( Supplementary Fig. 4b ). In addition, 8-OHdG content in heart and kidney DNA was measured. No difference between KO mice and controls was found in kidney DNA. However, in the heart of KO mice a significant reduction in 8-OHdG levels was observed ( Supplementary Fig. 4c ). Taken together, these findings suggest that despite a global deficit in UQ, aog Mclk1 KO mice do not suffer increased oxidative stress, even at a late stage in life. Changes in expression of antioxidant enzymes often occur in response to alterations in oxidative stress levels. Hence, we next looked at the steady-state levels of antioxidant enzymes in the kidneys and heart in which UQ depletion is most severe. Interestingly, we detected a lower level of the cytoplasmic superoxide dismutase 1 (SOD1) in kidney and heart at 6 months, as well as a markedly decreased level of catalase in kidneys ( Fig. 5b,c and Supplementary Fig. 5a ). We speculate these to be compensatory responses that may be induced by low cytoplasmic ROS and which help maintain ROS at physiological levels necessary for optimal cell function. The reduction in catalase levels could also be caused by a peroxisomal deficiency, given the known presence of UQ in peroxisomes and its requirement for peroxisome function [23] . We found no significant changes in SOD2 levels or activity in kidney mitochondria, but a mild decrease in SOD2 activity in heart mitochondria without an accompanying change in protein level ( Supplementary Fig. 5b,c ). From these observations, we conclude that the low levels of UQ in the cells of aog Mclk1 KO mice do not elevate oxidative stress in either the mitochondrial or cytoplasmic compartments. Dietary UQ supplementation fails to rescue aog Mclk1 KO mice To test whether UQ 10 supplementation could have beneficial effects for aog Mclk1 KO mice, the animals were given LiQsorb UQ 10 in the drinking water immediately after the last dose of TM. In a previous study, we observed that this easily absorbed form of UQ 10 can be taken up and used by the liver [9] . Here we found that UQ 10 treatment had only a minimal rescuing effect on aog Mclk1 KO mice. Overall, UQ 10 -treated mice were indistinguishable from untreated mice, with the same level of growth retardation after 6 months of UQ 10 feeding ( Fig. 6a ). Median survival time, however, was very slightly increased by the treatment, although not significantly ( Fig. 6b ). To determine whether dietary UQ 10 was actually taken up by the tissues, UQ quantification was carried out after 3 months of UQ 10 feeding. In both aog Mclk1 KO and control mice, a significant increase in UQ 10 levels was evident only in the liver, but not in heart, kidneys and skeletal muscles ( Fig. 6c ). 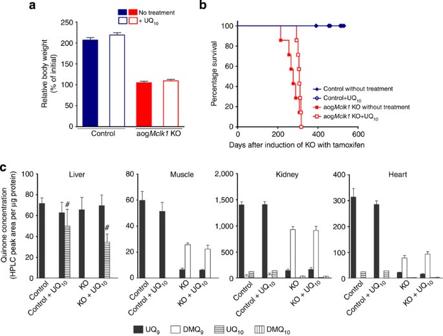Figure 6: Effects of UQ10supplementation on aogMclk1KO mice. UQ10was provided in drinking water after the last dose of TM (KO) or vehicle (control) to CAG-CreERT2;Mclk1loxP/loxPmice. (a) Comparison of body weights of UQ10-supplemented and not supplemented mice. Percentage changes in body weight after 6 months of UQ10treatment are shown. Values are percent weight relative to the initial weight at the beginning of the treatment. Error bars are s.e.m.n=7. (b) Effect of UQ10supplementation on the survival of aogMclk1KO mice. The KO mice fed UQ10showed a slight increase in median survival time (307 days) compared with the untreated KO group (277 days), but the difference was not statistically significant (n=7). (c) UQ levels after 3 months of UQ10supplementation. Columns indicate mean±s.e.m. of peak areas on HPLC chromatograms normalized to protein content (n=4).#P<0.001 versus untreated. As shown inFig. 3, a large depletion of UQ accompanied by an accumulation of DMQ was observed in the kidneys, heart and skeletal muscles of KO mice. Figure 6: Effects of UQ 10 supplementation on aog Mclk1 KO mice. UQ 10 was provided in drinking water after the last dose of TM (KO) or vehicle (control) to CAG- CreER T2 ;Mclk1 loxP/loxP mice. ( a ) Comparison of body weights of UQ 10 -supplemented and not supplemented mice. Percentage changes in body weight after 6 months of UQ 10 treatment are shown. Values are percent weight relative to the initial weight at the beginning of the treatment. Error bars are s.e.m. n =7. ( b ) Effect of UQ 10 supplementation on the survival of aog Mclk1 KO mice. The KO mice fed UQ 10 showed a slight increase in median survival time (307 days) compared with the untreated KO group (277 days), but the difference was not statistically significant ( n =7). ( c ) UQ levels after 3 months of UQ 10 supplementation. Columns indicate mean±s.e.m. of peak areas on HPLC chromatograms normalized to protein content ( n =4). # P <0.001 versus untreated. As shown in Fig. 3 , a large depletion of UQ accompanied by an accumulation of DMQ was observed in the kidneys, heart and skeletal muscles of KO mice. Full size image Rescue of UQ deficiency in aog Mclk1 KO mice by treatment with 2,4-DHB 2,4-DHB has previously been tested only on yeast deficient for the MCLK1 orthologue Coq7p (ref. 10 ). To establish whether 2,4-DHB could restore UQ synthesis in mammalian cells, we first treated Mclk1 KO fibroblasts [35] with the compound, which resulted in reappearance of UQ in these cells ( Supplementary Fig. 6 ). To treat mice, 2,4-DHB was added into the drinking water starting 2 weeks after completion of TM injections (when the KO was complete but the animals showed yet no sign of illness). Treated mice were characterized 6 months after KO induction. Striking differences were observed between treated and untreated mice. The KO mice on 2,4-DHB water were a lot heavier and looked much healthier than untreated aog Mclk1 KO controls ( Fig. 7a ), but remained lighter than animals that were never induced by TM ( Fig. 7b and Supplementary Fig. 7a ). Moreover, upon treatment, blood lactate levels were restored to the levels seen in control mice ( Supplementary Table 3 ), indicating a shift from high to low glycolytic rate. TG levels were simultaneously normalized ( Supplementary Table 3 ). Most strikingly, the survival of aog Mclk1 KO mice was markedly prolonged by the treatment ( Fig. 7c ). In fact, at the time of manuscript submission, treated mice have already been living twice as long as untreated and the oldest animals have already passed the age of 2 years. Except for their lower body weight, treated KO mutants are visually indistinguishable from the wild type. Interestingly, the treatment alone increased blood glucose, as shown by elevation of glucose concentrations in controls, as well as in those KO mice that were given a relatively higher dose of the precursor ( Supplementary Table 3 ). 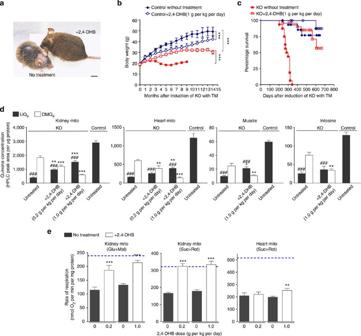Figure 7: Phenotypic rescue of aogMclk1KO mice by 2,4-DHB. (a) Representative image showing, at the same age, an untreated KO mouse and a KO mouse treated with 2,4-DHB (1 g kg−1of body weight per day) for~6 months. Scale bar, 1 cm. (b) Growth curves of 2,4-DHB-treated and untreated mice.n=6–14. ***P<0.001 (two-way analysis of variance (ANOVA)). (c) Kaplan–Meier survival curves of 2,4-DHB–treated and untreated mice.n=16–23. KO mice fed 2,4-DHB survived longer than untreated KO mice (P<0.0001). No effect was seen on controls (P=0.16). (d) Quinone levels in 2,4-DHB-treated aogMclk1KO mice.n=6–9. **P<0.01, ***P<0.001 compared with UQ9or DMQ9levels in untreated KO mice,###P<0.001 compared with UQ9concentrations in control mice (one-way ANOVA/Tukeypost hoctest). (e) State 3 mitochondrial respiration rates. Samples were the same as used ind.n=7–9. Blue dashed lines indicate the data for control mice (not induced by TM). Glu, glutamate; Mal, malate; Suc, succinate; Rot: rotenone. **P<0.01, ***P<0.001 compared with the untreated KO groups analysed on the same day (pairedt-test). All error bars are s.e.m. Figure 7: Phenotypic rescue of aog Mclk1 KO mice by 2,4-DHB. ( a ) Representative image showing, at the same age, an untreated KO mouse and a KO mouse treated with 2,4-DHB (1 g kg −1 of body weight per day) for~6 months. Scale bar, 1 cm. ( b ) Growth curves of 2,4-DHB-treated and untreated mice. n =6–14. *** P <0.001 (two-way analysis of variance (ANOVA)). ( c ) Kaplan–Meier survival curves of 2,4-DHB–treated and untreated mice. n =16–23. KO mice fed 2,4-DHB survived longer than untreated KO mice ( P <0.0001). No effect was seen on controls ( P =0.16). ( d ) Quinone levels in 2,4-DHB-treated aog Mclk1 KO mice. n =6–9. ** P <0.01, *** P <0.001 compared with UQ 9 or DMQ 9 levels in untreated KO mice, ### P <0.001 compared with UQ 9 concentrations in control mice (one-way ANOVA/Tukey post hoc test). ( e ) State 3 mitochondrial respiration rates. Samples were the same as used in d . n =7–9. Blue dashed lines indicate the data for control mice (not induced by TM). Glu, glutamate; Mal, malate; Suc, succinate; Rot: rotenone. ** P <0.01, *** P <0.001 compared with the untreated KO groups analysed on the same day (paired t -test). All error bars are s.e.m. Full size image 2,4-DHB treatment resulted in significantly increased but not wild-type UQ 9 levels in heart, kidneys and skeletal muscles ( Fig. 7d ). The increase in UQ 9 levels was accompanied by a lesser accumulation of DMQ 9 ( Fig. 7d and Supplementary Fig. 6 ). The same pattern was seen in the small intestine but the increase was not statistically significance. Polarographic measurements of respiration of heart and kidney mitochondria showed improvements of state 3 respiration, with the effect most evident in kidney mitochondria ( Fig. 7e ). Specifically, state 3 respiration in kidney mitochondria was almost completely restored by 2,4-DHB treatment, even at the relatively lower dose (0.2 g kg −1 body weight per day). In the heart, however, it was only at the higher dose (1 g kg −1 body weight per day) that a small, albeit significant, increase of state 3 respiration was observed ( Fig. 7e ). To verify that the levels of expression of Mclk1 had not changed in the treated aog Mclk1 KO mice, protein extracts were prepared from kidneys and analysed for the presence of MCLK1 by immunoblotting. As shown ( Fig. 2a ), loss of MCLK1 expression was maintained 6 months after the last TM administration and was not at all affected by treatment with 2,4-DHB. Thus, as expected, treating aog Mclk1 KO mice with 2,4-DHB rescues disease phenotypes and extends lifespan without restoring MCLK1 levels. Intriguingly, dietary 2,4-DHB also appears to have an effect on control mice (that is, CAG -CreER T2 ;Mclk1 loxP/loxP mice not induced by TM). As shown ( Fig. 7b and Supplementary Fig. 8a,b ), the control mice treated with 2,4-DHB gained less body weight than untreated mice. Except for this, we observed no phenotypic abnormalities in the treated mice ( Fig. 7c and Supplementary Fig. 8a ). To explore if the weight loss resulted from 2,4-DHB interfering with UQ metabolism, we treated controls with a higher concentration of 2,4-DHB (2.5 g kg −1 body weight per day) and for a longer time (~10 months). This resulted in both weight loss and changes in UQ levels, including a paradoxical elevation in the kidney and moderate losses in heart, liver and muscle but without effects on mitochondrial function ( Supplementary Fig. 8b–d ). It remains unclear, therefore, which aspect of UQ function induces weight loss upon treatment with 2,4-DHB in animals with intact UQ biosynthesis. UQ deficiency-induced phenotypes are reversible To determine whether the phenotypes produced by loss of UQ are reversible, one cohort of aog Mclk1 KO mice was not immediately treated with 2,4-DHB but only 6 months after TM induction, a time point when untreated KO mice already displayed severe phenotypes. This late-onset treatment was nonetheless able to successfully rescue the KO mice. As shown ( Fig. 8a ), after 2 months on 2,4-DHB, the late-treated KO mice already showed a marked improvement in overall health. They regained body weight, grew back lost fur and outwardly became normal-looking. Furthermore, the treatment even allowed KO mice to resume a normal lifespan ( Fig. 8b ). In fact, these mice had a median lifespan of ~2.1 years, which is statistically indistinguishable from that of the control mice subjected or not to the same treatment ( Fig. 8b ). Even at old age, mutant mice rescued by late-onset treatment appeared phenotypically indistinguishable from the wild type expect for a slightly leaner appearance ( Fig. 8c ). In addition, similar to the effect of treatment started immediately after the KO, we observed that 8 months after the beginning of late-onset treatment, basal lactate levels were indistinguishable from age-matched controls, despite the fact that UQ levels in some major tissues were still considerably lower than normal (<30% of control levels; Supplementary Fig. 9a,c ). Mean BUN levels were also comparable in the two groups of mice, indicating minimal or no renal functional deficit ( Supplementary Fig. 9b ). 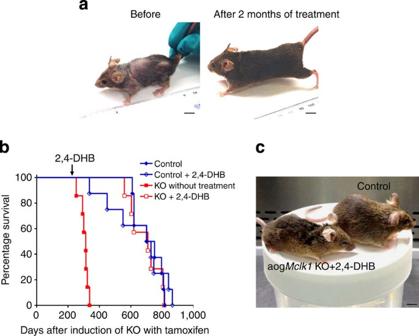Figure 8: Effect of late treatment of aogMclk1KO mice treatment with 2,4-DHB. Mice were given 2,4-DHB (1 g/kg body weight/day) from~6 months after the last dose of TM or vehicle. (a) A representative picture of KO mice before the start and after 2 months of treatment. (b) The late treatment significantly extended the survival of aogMclk1KO mice (P<0.001 versus untreated KO group; log-rank test). No significant difference in lifespan was observed between treated KO mice and control mice (P=0.62).n=7–8. (c) A representative picture of KO mice after ~17.5 months of 2,4-DHB treatment started 6 months after the KO in comparison with an age-matched control (not induced by TM). Scale bars, 1 cm. Figure 8: Effect of late treatment of aog Mclk1 KO mice treatment with 2,4-DHB. Mice were given 2,4-DHB (1 g/kg body weight/day) from~6 months after the last dose of TM or vehicle. ( a ) A representative picture of KO mice before the start and after 2 months of treatment. ( b ) The late treatment significantly extended the survival of aog Mclk1 KO mice ( P <0.001 versus untreated KO group; log-rank test). No significant difference in lifespan was observed between treated KO mice and control mice ( P =0.62). n =7–8. ( c ) A representative picture of KO mice after ~17.5 months of 2,4-DHB treatment started 6 months after the KO in comparison with an age-matched control (not induced by TM). Scale bars, 1 cm. Full size image Six months after the induction of the KO, we observed that a severe depletion of UQ (down to ~10% of normal UQ levels) in the heart, kidneys and skeletal muscles produced a marked (50%) decline in mitochondrial state 3 respiration ( Fig. 4a,b ). This is in contrast to what we had previously found using a murine model of liver-specific MCLK1 loss, where a similarly large depletion of UQ in hepatocytes caused only a mild impairment of respiratory chain function, consistent with what has been found with liver-specific Pdss2 ablation [9] , [40] . However, we also found that state 3 respiration was fully restored in kidney mitochondria from 2,4-DHB-treated aog Mclk1 KO mice, despite UQ levels that were still <35% of normal ( Fig. 7d,e ), suggesting that the kidney, as the liver, produces UQ in amounts in excess of those required to sustain normal mitochondrial respiratory chain function. This is in contrast to heart mitochondria, where a partial rescue of UQ biosynthesis, reaching ~35% of the wild-type level, resulted in only a small increase in state 3 respiration compared with untreated KO controls ( Fig. 7d,e ). Thus, compared with kidney and liver, the heart appears to have a lower UQ reserve for mitochondrial respiration. Surprisingly, total oxygen consumption as measured by indirect calorimetry was higher in aog Mclk1 KO mice than in control mice ( Supplementary Fig. 1c ). These animals are small and almost devoid of subcutaneous fat. Thus, one possibility is that the increased oxygen consumption is the result of mitochondrial uncoupling, which could be an adaptive change to increase heat production in order to maintain core body temperature. This would have to result from a regulated in vivo adaptation, given that in isolated heart and kidney mitochondria from KO mice the ADP/O ratio was not significantly changed ( Supplementary Table 1 ). Elevated blood lactate levels in aog Mclk1 KO mice are consistent with the partially deficient mitochondrial oxidative metabolism that often results in an increase in glycolytic activity ( Table 1 ). In fact, lactic acidosis is a common symptom in patients with mitochondrial diseases including primary UQ deficiency [6] . In 2,4-DHB-treated aog Mclk1 KO mice, rescue of UQ production and hence of respiratory deficiency was accompanied by normalization of blood lactate ( Fig. 7d,e and Supplementary Table 3 ). This reflects a switch back to aerobic respiration. Glucose levels were decreased in KO mice, probably owing to a higher rate of glucose utilization ( Table 1 ). In addition, we observed that circulating TG levels were significantly lower in KO mice than in control mice, which could be a consequence of their severe loss of fat tissue given that (1) adipose tissue is a site of TG synthesis and storage, and (2) the liver, the central organ of TG metabolism, was not affected in KO mice. In agreement with this, weight gain after 2,4-DHB feeding, including fat deposition, was accompanied by restoration of TG levels to the normal range ( Supplementary Table 3 ). aog Mclk1 KO animals appeared to gradually deteriorate during 6 six months following KO induction, with weight loss, loss of coat hair and a frequently hunched posture, but it is not known for which reason they die several weeks later. However, at 6 months their behaviour, level of spontaneous activity and food consumption were still normal ( Fig. 2d,f and Supplementary Fig. 1d ), indicating that they were not suffering from acute organ failure. Thus, many tissues, including vital organs such as heart, kidney and skeletal muscles needed for basic vital functions such as heartbeat, breathing, feeding and waste elimination, appear to function sufficiently well with only half of their mitochondrial respiratory capacity. Furthermore, the fact that echocardiography showed no obvious cardiac abnormalities ( Supplementary Fig. 2 ), and that although feeding 2,4-DHB only minimally rescued cardiac mitochondrial function ( Fig. 7e ), the treatment was sufficient to extend lifespan markedly ( Figs 7c and 8b ) suggest that cardiomyocytes have a remarkably long-term tolerance to low mitochondrial respiratory capacity. This is surprising, given the well-known function of UQ in the ETC and the high-energy expenditure of the cardiac muscle, which depends almost entirely on the high mitochondrial content of cardiomyocytes. Further studies will be needed to understand how this is possible despite the well-studied links between heart disease and mitochondrial dysfunction. A variety of mouse models of mitochondrial dysfunction have previously been described. They use genetic ablation of protein subunits of ETC complexes, ETC complex assembly factors or genes required for mitochondrial maintenance [25] , [41] , [42] , [43] , [44] . For most of them, even tissue-specific conditional KOs exhibit progressive severe mitochondrial disease, much worse than what we describe for aog Mclk1 KO mice [45] , [46] , [47] , [48] . A number of factors might contribute to explain why aog Mclk1 KO mutants have a relatively mild phenotype: mitochondrial dysfunction is induced only at the adult stage, they display no sign of increased oxidative stress, the loss of UQ is gradual and low UQ might result in slow but, possibly, not abnormal or otherwise impaired electron transport. UQ is well recognized as a superoxide generators in the ETC, as the ubisemiquinone radicals (SQ ·− ) generated during mitochondrial electron transport are thought to be capable of prematurely donating their electrons to oxygen, thereby resulting in the formation of superoxide. The SQ ·− formed at the Q o site of complex III is an important source of ROS [3] . However, it is less clear whether at complex I the UQ site also contributes or whether superoxide is produced from the reduced flavin alone [4] . In the present study, we showed that when respiring on complex I substrates, UQ-deficient heart mitochondria from aog Mclk1 KO mice show a lower rate of H 2 O 2 production in the presence of rotenone ( Fig. 5a ). This observation supports the idea that at complex I, SQ ·− species also play a role as superoxide generators. Indeed, if they did not, the blockage of electron flow through the UQ-binding site by rotenone, which maximizes the reduction of the upstream redox groups (including the flavin site), should not give different rates of superoxide production in UQ-abundant and UQ-depleted mitochondria. Reduced H 2 O 2 production in the mutant mitochondria when succinate is the substrate and the attenuation of H 2 O 2 production by rotenone are consistent with the model of reverse electron transport, which describes that the backflow of electrons into complex I through the UQ-binding site(s) mainly accounts for ROS generation in succinate-energized mitochondria [49] . Finally, in the presence of antimycin A, the heart mitochondria from KO mice were found to produce H 2 O 2 at a much lower rate than normal controls ( Fig. 5a ), consistent with SQ ·− being the source of electron leakage from complex III (ref. 3 ). The earliest reports on an antioxidant function of UQ date back to a half-century ago. The strongest evidence came from studies with crude submitochondrial preparations, which showed that the addition of NADH or succinate can reduce oxidative damage (presumably by generating more reduced UQ) and the protective effect was abolished on removal of bulk UQ [50] . Besides the mitochondria, UQ is also present in the plasma membrane and other intracellular membranes of eukaryotic cells where it is thought to protect these structures as well from oxidative stress [5] . UQ has been one of the most popular anti-ageing supplements, mainly based on the logic that more UQ may help the body fight oxidative stress. In addition, UQ levels have been reported to decline with advancing age [50] , although it could not be established whether this has clinical significance. We could not demonstrate increased oxidative damages in aog Mclk1 KO mice, which showed normal levels of plasma F 2 -isoprostanes and 8-OHdG 8 months after disruption of UQ biosynthesis ( Supplementary Fig. 4a,b ). Moreover, no increased DNA oxidative damage (8-OHdG) was detected in the kidneys and heart with only 10% of the normal UQ concentration ( Supplementary Fig. 4c ). These normal levels of oxidative damage were not the result of any upregulation of antioxidant enzymes, as the expression levels of SOD1, catalase and SOD2 were found be either indistinguishable from controls or even significantly lower ( Fig. 5b,c and Supplementary Fig. 5 ). Thus, we show here for the first time that severe UQ deficit in vivo does not cause an elevated level of oxidative stress. This result is consistent with in vitro findings in fibroblasts from primary UQ deficiency patients [51] . The overall oxidative stress in aog Mclk1 KO mice is the net result of the effects of UQ deficit on the level of ROS production and elimination. We demonstrate that the H 2 O 2 production rates are lower in the heart mitochondria from KO mice as compared with controls with intact UQ content ( Fig. 5a ). It is possible that in the cells of aog Mclk1 KO mice decreased antioxidant activity of UQ is exactly balanced out by less mitochondrial ROS production. However, given that in the KO cells mitochondrial respiration is two times lower than normal, but UQ content is up to ten times lower, we think that this is unlikely. Rather, the data suggest that UQ is not crucial to keep oxidative stress low. This does not exclude that UQ could be required as antioxidant in vivo in particular pathological situations. Similarly, it is possible that UQ might have beneficial pharmacological activities when used as a supplement. However, such activities would likely be unrelated to the size of the intracellular pool of UQ, given our observation that supplemented UQ does not enter most tissues and cannot rescue the phenotype of aog Mclk1 KO mice. We found that feeding ago Mclk1 KO mice with 2,4-DHB even after they were already severely ill and only weeks away from death could restore a healthy phenotype, including a normal lifespan ( Fig. 8 ). Given the vital role of UQ in ETC function and the great importance of mitochondria in health and disease [2] , [52] , it is reasonable to think that 2,4-DHB rescues the lethal phenotype of ago Mclk1 KO mutants mainly by restoring mitochondrial respiratory function. Given that the treatment restores a normal lifespan, one can further postulate that the pathophysiological alterations that cause the shortened survival of the ago Mclk1 KO mice (median survival ~9 months) are effectively corrected after reestablishment of proper ETC function. However, this is a striking finding because mitochondrial dysfunction is believed by many to be central to the biology of ageing and the pathogenesis of age-related diseases [53] . It has repeatedly been suggested that the OXPHOS deficiency, aberrant production of ROS and increased mtDNA mutations that occur with increasing age cause irreparable cell damage, leading to the irreversible degenerative processes that accompany ageing and ultimately result in death [54] , [55] , [56] . Although the cause of the mitochondrial dysfunction in our model (UQ deficiency) is different from those observed during normal ageing, our observations are nonetheless incompatible with the classical viewpoint. Indeed, if mitochondrial dysfunction were causal to ageing, we would expect that the mitochondrial dysfunction sustained in ago Mclk1 KO mice before treatment with 2,4-DHB to have produced irreversible degenerative secondary pathologies, and thus that these mice should still have shortened lifespan even after treatment, which is not what we observe. More than 20 distinct pathogenic mutations in seven different UQ biosynthetic genes have been identified in patients since 2006 (refs 6 , 11 , 12 , 13 , 14 , 15 , 16 , 17 , 18 , 19 ). In addition, secondary UQ deficiencies due to mutations in other genes including in mtDNA are frequently observed in patients with mitochondrial disease syndrome [57] , [58] . To date, the only available treatment for the disease is UQ supplementation, but its efficacy is variable and limited, presumably because of very poor uptake by most tissues except the liver [13] , [14] , [15] , [17] , [19] , [59] , [60] , [61] . The robust phenotypic rescue of aog Mclk1 KO mice by 2,4-DHB feeding demonstrates that animal cells can readily take up this compound from dietary sources and use it as a biosynthetic precursor of UQ. All enzymes upstream of MCLK1 appear capable of acting relatively efficiently on this unnatural substrate and its metabolites. We also found that the elevation in UQ levels following 2,4-DHB treatment was coupled with decreased production of DMQ ( Fig. 7d and Supplementary Fig. 6 ), suggesting a partial suppression of the native UQ biosynthetic pathway in which 4-HB normally serves as the precursor of the UQ benzoquinone ring. This is most likely due to competition between 4-HB and 2,4-DHB and their metabolites for access to the catalytic sites of the COQ enzymes upstream of MCLK1 ( Fig. 1a ). This notion could also explain decreased level of UQ in control mice after long-term feeding of 2,4-DHB ( Supplementary Fig. 8c ). When acting on the unnatural substrate and its metabolites, COQ enzymes likely work less efficiently than with 4-HB and the natural intermediates, and, therefore, cells in which both precursors participate in UQ biosynthesis produce a lower than normal level of UQ. Our findings that UQ 10 supplementation was mostly ineffective at rescuing aog Mclk1 KO mouse mutants, but that 2,4-DHB can markedly rescue mutant pathological phenotypes, may have important clinical implications ( Figs 6 , 7 , 8 ). Specifically, they substantiate the idea that manipulations of a defective UQ biosynthetic pathway with hydroxylated analogues of 4-HB could benefit patients with some types of primary UQ deficiency. Although no patients with defects in COQ7 have yet been identified, several independent pathological mutations in COQ6 have been described in UQ-deficient patients [17] . This is of interest because studies in yeast have shown that loss of Coq6p can be bypassed by providing the precursor 3,4-DHB [62] , [63] , a situation parallel to that described here for MCLK1/COQ7. Furthermore, a patient with a COQ9 mutation who died at 2 years of age despite UQ 10 therapy has been described [18] . Although the exact role of COQ9 in the biosynthesis of UQ is not understood, mutant phenotypes in a Coq9 mouse model indicate that loss of COQ9 impairs UQ biosynthesis by reducing MCLK1/COQ7 activity [64] . Thus, 2,4-DHB could have therapeutic potential for treating COQ9 patients. It is very likely that patients would very well tolerate the hydroxylated analogues of 4-HB, even at high concentrations. Indeed, both of them, especially 2,4-DHB, have been used as food flavour modifiers because of their sweet taste and ability to enhance the sweetness delivery of other artificial sweeteners. In fact, 2,4-DHB is present in a broad range of food products and drinks, such as beverages, fish products, snack foods and chewing gums. One case report where 2,4-DHB was administered to patients with rheumatic fever described that no severe side effects were seen at the oral dose of 5,330–6,000 mg per day for up to 16 days [65] . An important first step to explore the potential use of 4-HB analogues in treatment of human disease would be to test the effects of such treatments on mouse mutants that carry mutations that are analogous to those found in human patients. Considering that there is still some residual biosynthesis of UQ in human patients [17] , [18] and our observation of inhibition of the native UQ biosynthetic pathway in the presence of 2,4-DHB, the possible aggregated effects of bypass and inhibition need to be addressed carefully. Our results suggest that using ‘bypass’ precursors could be a promising new therapeutic approach for enzymatic defects in biosynthetic pathways. Numerous inborn single gene diseases or disease predispositions are the result of enzymatic deficiency in biosynthetic pathways [66] . The disease phenotypes can result from the absence of an essential metabolite or the production and accumulation of toxic intermediates. Some disease can be alleviated by providing the missing product such as defects in bile acid synthesis [67] or in tyrosine hydroxylase [68] . In others, such as classic phenylketonuria, relief is obtained by minimizing the activity of the pathway by starving it of substrate, in this case phenylalanine [69] . Our findings suggest that there would be value in exploring more systematically a third approach that consists in providing an alternative bypass precursor that incorporates chemical groups that are normally provided to the end product by the deficient enzymatic step. This approach might have additional benefits when the intermediates that accumulate are toxic, as a bypass precursor might successfully compete with the natural precursor to lower the levels of toxic intermediate, similar to what we have observed for DMQ ( Fig. 7d ). Mice Conditional Mclk1 -floxed mice [9] were crossed to CAG- CreER T2 mice (The Jackson Laboratory), and Cre-mediated excision was induced in 6–8-week-old CAG- CreER T2 ;Mclk1 loxP/loxP female mice by injection with TM (6 mg kg −1 body weight for a total of eight injections every other day) intraperitoneally. Females of the same genotype injected with vehicle alone (corn oil) were used as controls. Mice used were on a mixed Sv129/C57BL/6 background. Unless otherwise stated, experiments were performed on female mice 6 months after the last TM or vehicle administration. For treatment experiments, 2,4-DHB (Sigma, 0.2–2.5 g kg −1 body weight per day) or UQ 10 (LiQsorb, ~300–400 mg kg −1 body weight per day) was added to the drinking water. Care of mice followed the guidelines of the Canadian Council on Animal Care and all the procedures were approved by the Animal Care and Use Committee of McGill University. Genotyping primers are provided in Supplementary Table 4 . Identification and quantification of quinones Quinones were extracted with a mixture of ethanol and hexane as previous described [9] . Briefly, tissue homogenates or mitochondria were mixed with an equal volume of hexane/ethanol for 10 min by vortexing, centrifuged for 5 min at 8,000 g and the hexane layer was collected. After evaporation to dryness using a vacuum centrifuge, the quinone residue was dissolved in ethanol and stored at −20 °C until HPLC analysis. A Beckman System Gold HPLC with a reversed-phase C18 column (5 μm, 4.6 × 250 mm) was used. The mobile phase was 70% methanol and 30% ethanol at a flow rate of 1.8 ml min −1 . The ultraviolet detector was set at 275 nm. UQ 6 was used as an internal standard to correct for extraction efficiency. Total quinone levels were normalized to protein content. Mitochondria isolation and respiration measurements Mitochondrial isolation was performed using standard homogenization and differential centrifugation methods similar to previous studies [9] , [70] . Each fresh heart was homogenized with a Polytron tissue disruptor (Power Gen 125, Fisher Scientific) in a buffer containing 70 mM sucrose, 220 mM mannitol, 1 mM EGTA, 0.1% fatty acid-free bovine serum albumin (BSA), and 10 mM HEPES, pH 7.4. Kidneys were immersed in an isolation buffer consisting of 250 mM sucrose, 1 mM EDTA and 10 mM HEPES buffer, pH 7.4, minced with scissors and then homogenized with a motor-driven Teflon Potter-Elvehjem homogenizer (Wheaton, Millville, NJ). For isolation of muscle mitochondria, mixed gastrocnemius muscles were placed into an isolation buffer containing 100 mM sucrose, 46 mM KCl, 10 mM EDTA and 100 mM Tris-base, pH 7.4, and minced with scissors after addition of the protease Nagarse (at 10% (v/v)). After 5 min incubation on ice, minced muscle was pipetted out, re-suspended in 10 ml of the isolation buffer and then homogenized using a Teflon Potter-Elvehjem homogenizer. To collect mitochondria, tissue homogenates were first subjected to low-speed centrifugation (700 g ) for 10 min. The resultant supernatant was then centrifuged for 10 min at 10,000 g (Beckman Coulter Avanti J-25) to pellet mitochondria. After washing once, the final pellet was re-suspended in a small volume of the same isolation buffers. All steps were performed at 4 °C or on ice. Freshly isolated mitochondria were used immediately for measuring oxygen consumption, and the remaining was frozen and stored at −80 °C for western blots and enzymatic activity assays. Mitochondrial respiration was measured using the OROBOROS Oxygraph-2k at 30 °C (Oroboros Instruments). The respiration media contained 0.5 mM EGTA, 3 mM MgCl 2 .6H 2 O, 60 mM potassium lactobionate, 20 mM taurine, 10 mM KH 2 PO 4 , 20 mM HEPES, 110 mM sucrose, and 1 g l −1 fatty acid-free BSA, pH 7.1. To measure complex I-mediated respiration, the combination of 5 mM glutamate/2.5 mM malate was used as substrates. Succinate (10 mM) plus rotenone (1.25 μM) was used to quantify complex II-dependent respiration after blocking backflow into complex I. State 3 respiration was recorded after adding ADP to a final concentration of 0.6 mM. State 4 respiration was determined as the rate of oxygen consumption after exhaustion of ADP. Data are expressed as nmoles oxygen consumed per min per mg protein. The respiratory control ratio was given by state 3/state 4 respiration. The ADP/O ratio was calculated as the amount of added ADP (in nmoles) divided by the amount of oxygen atoms consumed during state 3 respiration. Assays for the activities of respiratory chain complexes The activities of mitochondrial respiratory complexes I-III, II-III, I, II and III were measured using previously described methods [9] , [70] . All assays were carried out spectrophotometrically at 30 °C using a double-wavelength Beckman DU 640 spectrophotometer. The activities of complex I-III and complex II-III were measured by following the reduction of cytochrome c at 550 nm in the presence of complex I (NADH) or II (succinate) substrate, respectively. The complex I-III assay was performed in a buffer containing 25 mM potassium phosphate (pH 7.4), 0.1 mM NADH and 2 mM KCN. The reaction buffer for the complex II-III activity assay consisted of 25 mM potassium phosphate (pH 7.4), 20 mM succinate, 2 μg ml −1 rotenone, 0.5 mM EDTA and 2 mM KCN. In order to fully activate complex II, reaction mixtures were pre-incubated at 30 °C for 10 min after addition of mitochondria. After addition of mitochondria (10–20 μg ml −1 ) and cytochrome c (30 μM), OD550 was recorded at 30 s intervals over 5 min in the presence or absence of a specific ETC inhibitor (that is, 5 μg ml −1 rotenone for the complex I-III assay and 10 mM malonate for the complex II-III assay). The extinction coefficient 19.1 mM −1 cm −1 was used for cytochrome c . For the complex I assay, mitochondria were added to a potassium phosphate buffer (25 mM, pH 7.4) containing 3.5 g/l defatted BSA, 2 mM KCN, 2 μg ml −1 antimycin A, 0.1 mM UQ 1 and 0.1 mM NADH. NADH oxidation was then monitored at 340 nm in the absence or presence of rotenone (2 μg ml −1 ). The extinction coefficient for NADH used was 6.81 mM −1 cm −1 . Complex II activity was assayed by following the reduction of dichlorophenolindophenol (DCPIP; 0.15 mM) at 600 nm in a buffer composed of 25 mM potassium phosphate (pH 7.4), 20 mM succinate, 2 μg antimycin A, 2 μg rotenone, 0.1 mM UQ 1 and 2 mM KCN. The DCPIP reduction rate was calculated using an extinction coefficient of 21 mM −1 cm −1 , and the background rate for non-enzymatic reduction of DCPIP was corrected by subtracting the values obtained in the presence of 20 mM malonate. Complex III activity was measured by following the reduction of cytochrome c at 550 nm in the presence of decylubiquinol as a substrate. The reaction medium was 25 mM potassium phosphate buffer (pH 7.4) supplemented with 1 mM KCN, 4 μg ml −1 rotenone, 50 μM cytochrome c , 60 μM decylubiquinol and 0.1% BSA. Decylubiquinol was prepared by reducing decylubiquinone with sodium dithionite. The reaction was started with 25 μg of mitochondrial protein and sensitivity to a mixture of complex III inhibitors (10 μg ml −1 antimycin A+2 μg ml −1 of myxothiazol) was used as a measure of complex III-specific activity. Specific ETC enzyme activities are calculated by subtraction of values obtained in the presence of specific complex inhibitors and are finally expressed as nmoles of electron acceptor reduced per min per mg mitochondrial protein. The Bradford assay was used to quantify the protein concentration. Measurement of CS activity CS activity was determined by the rate of DTNB (5, 5′-dithio-bis [2-nitrobenzoic acid]) reduction, which is coupled with citrate formation catalysed by CS at 412 nm. Reaction mixtures contained 100 mM Tris (pH 8.0), 0.1% Triton X-100, 0.1 mM acetyl-CoA, 0.1 mM DTNB and 0.25 mM oxaloacetate. Activities were calculated as nmol of citrate formed per min per mg of protein using an extinction coefficient of 13.6 mM −1 cm −1 . Mitochondrial H 2 O 2 production rates ROS production by heart mitochondria was measured using an adapted Amplex Red/HRP method [70] . Heart mitochondria (0.2 mg ml −1 ) were incubated in assay medium (125 mM KCl, 2 mM KH 2 PO 4 , 10 mM HEPES, 2 mM MgCl 2 , 0.2 mM EGTA and BSA 0.1% (w/v), pH 7.2) containing 50 μM Amplex Red, 5 units per ml HRP and 20 units per ml superoxide dismutase. The increase in Amplex Red fluorescence was followed over 10 min at 30 °C at 545/590 nm in a microplate reader (TECAN Infinite 200). ROS production was initiated by the addition of a mixture of glutamate (10 mM) and malate (5 mM) or succinate (10 mM) in the presence or absence of rotenone (10 μM) and/or antimycin A (5 μg ml −1 ). Arbitrary fluorescence was converted to known amounts of H 2 O 2 using standard curves prepared on the same day. Results are expressed as nmoles of H 2 O 2 per min per mg of mitochondrial protein. Locomotory activity Physical activity was measured using a comprehensive laboratory animal monitoring system (Columbus Instruments). Mice were housed individually with free access to food and water. The X-total count (X-TOT) that records any horizontal movement >0.5 inch was monitored for 2 days after an acclimation period of at least 3 h. Blood and plasma measurements Blood glucose levels were measured from a drop of blood obtained from the tail vein using a commercial glucometer (ACCU-CHEK Aviva) after overnight fasting. Tail blood lactate concentrations were determined using a lactate meter (Lactate Plus) in resting mice. Blood glucose was measured every week for 3–4 weeks and a mean value was obtained for each individual mouse. Lactate measurement was done twice with an interval of 1 week. The Infinity Triglyceride reagent kit (Thermo Scientific) was used to determine plasma triglyceride levels. Immunoblotting For western blotting analysis of MCLK1, crude mitochondrial lysates were separated on 12% SDS–PAGE gels and transferred onto polyvinylidene fluoride membranes (Bio-Rad). Membranes were blocked with 5% non-fat milk in PBS and probed overnight at 4 °C, with a polyclonal antibody against MCLK1 (1:500, rabbit polyclonal; developed in our laboratory) [8] . The protein loading was monitored with an anti-porin antibody (1:2,000, mouse monoclonal; Abcam). After three washing steps with PBS 0.05% Tween 20, the membranes were incubated with HRP-coupled secondary anti-mouse (1:10,000; Pierce) and anti-rabbit (1:2,000; Sigma) antibodies at room temperature for 2 h. The membranes were developed with ECL plus detection reagent (GE Healthcare) and the chemifluorescent signal was visualized using a Typhoon 9400 scanner (GE Healthcare). Western blotting of SOD1 and catalase were performed with total protein extracts from mouse tissues prepared in radio-immunoprecipitation assay buffer (50 mM Tris HCl, 150 mM NaCl, 1.0% NP-40, 0.5% sodium deoxycholate and 1.0 mM EDTA, pH 7.4) containing protease inhibitors. Equal amounts of total protein (20–40 μg) were separated by electrophoresis on 12% SDS–PAGE gel and then immunoblotted with anti-SOD1 (1:2,000, Abcam) or anti-catalase (1:2,000, Abcam) antibody. As loading controls, α-tubulin (1:1,000; Cell Signaling Technology) and β-actin (1:1,000; Cell Signaling Technology) were used. Blots were developed using ECL reagents (GE Healthcare) and exposed to CL-XPosure film (Pierce). Band densities were quantified using Thermo Scientific myImageAnalysis software. Statistical analysis Results are presented as mean±s.e.m. The sample sizes used were based on the variability expected and previous experience. In experiments involving animals, there were no exclusions. No randomization methods were used. Differences between survival curves were evaluated with the log-rank test. All time-course data were analysed using a two-way analysis of variance (ANOVA) coupled with a Bonferroni post hoc test. For all other variables, Student's t -test or one-way analysis of variance with Tukey’s post hoc test was used as appropriate. Differences of P <0.05 were considered significant. How to cite this article: Wang, Y. et al . Mitochondrial function and lifespan of mice with controlled ubiquinone biosynthesis. Nat. Commun. 6:6393 doi: 10.1038/ncomms7393 (2015).